Quantitative maps of protein phosphorylation sites across 14 different rat organs and tissues Deregulated cellular signalling is a common hallmark of disease, and delineating tissue phosphoproteomes is key to unravelling the underlying mechanisms. Here we present the broadest tissue catalogue of phosphoproteins to date, covering 31,480 phosphorylation sites on 7,280 proteins quantified across 14 rat organs and tissues. We provide the data set as an easily accessible resource via a web-based database, the CPR PTM Resource. A major fraction of the presented phosphorylation sites are tissue-specific and modulate protein interaction networks that are essential for the function of individual organs. For skeletal muscle, we find that phosphotyrosines are over-represented, which is mainly due to proteins involved in glycogenolysis and muscle contraction, a finding we validate in human skeletal muscle biopsies. Tyrosine phosphorylation is involved in both skeletal and cardiac muscle contraction, whereas glycogenolytic enzymes are tyrosine phosphorylated in skeletal muscle but not in the liver. The presented phosphoproteomic method is simple and rapid, making it applicable for screening of diseased tissue samples. Protein phosphorylation is a post-translational modification implicated in a diverse variety of cellular processes, spanning from proliferation and differentiation to apoptosis. Site-specific phosphorylation events can function as molecular switches that either activate or inhibit protein activity, dictate sub-cellular localization or act as recruitment platforms for interacting proteins with special domains (such as SH2, PTB, BRCT, 14-3-3 and FHA domains). Cellular protein phosphorylation is tightly controlled by protein kinases and phosphatases, and as these enzymes have differential expression levels across tissues, protein phosphorylations are dynamic events with restricted spatial and temporal distribution. The activity of kinases and phosphatases are themselves fine-tuned by phosphorylation events, thereby interconnecting signalling pathways outlining a complex regulatory pattern. Phosphorylation events have been implicated in the pathophysiology of several severe diseases, such as cancer, diabetes and neuropsychiatric disorders [1] , [2] , [3] , [4] , [5] , [6] . For instance, in leukemia, activating mutations in kinases such as flt3 (ref. 7 ) and bcr-abl [8] are often the oncogenic drivers of cell transformation. The fact that deregulated signalling is a hallmark of many diseases highlights the importance of developing techniques that allow for rapid, comprehensive and quantitative determinations of tissue phosphoproteomes. Quantitative mass spectrometry (MS)-based phosphoproteomics is currently the most powerful technique for analysis of cellular signalling networks [9] . Advances of the methodology have mainly been driven by the introduction of robust methods for phosphopeptide enrichment [10] , [11] , [12] in combination with stable isotope labelling techniques [13] , [14] and high-resolution hybrid mass spectrometers [15] . We and others have previously described methods to study global phosphorylation site changes as a function of specific stimuli [16] , [17] , [18] , [19] . However, these investigations were typically the results of huge efforts requiring hundreds of hours of mass spectrometric analysis and were all conducted in cell lines. So far, there have only been limited attempts to analyse phosphoproteomes of tissues and organs on a systems-wide scale [20] , [21] , [22] , [23] . Such attempts have all been based on extensive fractionation by ion-change chromatography to reduce sample complexity and low-resolution tandem MS, necessitating days of mass-spectrometric measurement time per tissue sample. Rodent models exist for many human signalling diseases and to date phosphoproteomes of nine mouse tissues has been analyzed in-depth [20] . However, the rat has important advantages relative to mouse for the study of cardiovascular diseases, diabetes, arthritis and many autoimmune, neurological, behavioural and addiction disorders [24] as well as for testing pharmacodynamics and toxicity of potential therapeutic compounds [25] . Therefore, we aimed to quantify the rat organ phosphoproteome in an in-depth and reproducible manner. Here we quantitatively map phosphoproteomes of 14 rat tissues and present a large data set of 31,480 phosphorylation sites from 7,280 proteins as a resource to the scientific community. We combine an effective tissue phosphoproteome preservation and homogenization protocol with a simple, single-step phosphopeptide enrichment method followed by higher-energy collisional dissociation (HCD) fragmentation [26] on an LTQ-Orbitrap Velos instrument [27] . This approach allows for in-depth investigation of tissue phosphoproteomes in single-shot liquid chromatography (LC)-MS analyses using a gradient of just 3 h, thus significantly reducing the time required for determination of a tissue phosphoproteome. In addition, HCD provides higher data quality covering the full mass region without a low-mass cut-off combined with high-resolution and accurate mass fragment ion measurements, which makes it a potent fragmentation technique for phosphopeptides [28] . Further underscoring the general applicability and translational aspects of the developed method, we validate the rat skeletal muscle phosphoproteome in human skeletal muscle biopsies. For each tissue, we systematically analyse the physical interactions of phosporylated proteins in silico to generate first drafts of spatial molecular networks regulated by tissue-specific phophatase and kinase dynamics. Phosphoprotein identification from 14 rat tissues To investigate phosphoproteins across tissues, organs were harvested from Sprague Dawley albino rats (Crl:SD) and they were all immediately snap frozen. We pooled organs from four rats to account for biological variation. The tissues isolated were: brain (dissected into cerebellum, cortex and brainstem), heart, muscle, lung, kidney, liver, stomach, pancreas, spleen, thymus, perirenal fat, intestine, testis and blood ( Fig. 1 ). To preserve the in-vivo state of the phosphoproteome and reduce post-mortem effects in dissected tissue samples, we eliminated endogenous enzymatic activity by thermal protein denaturation of the snap frozen samples using a Stabilizor T1 (Denator, Sweden). This procedure effectively abolish the activity of protein phosphatases, kinases, proteases and other enzymes that can change the protein modification site abundance during sample handling [29] . Next, we carefully homogenized the tissues in a urea buffer using ceramic beads on a Precellys 24 (Bertin Technologies, France). Following brief sonication, protein concentration was determined and from each tissue extract 10 mg protein was digested in solution with endoproteinase Lys-C and trypsin. Two rounds of phosphopeptide enrichment by titanium dioxide chromatography were performed, and the enriched phosphopeptide fractions were analysed by 3 h LC-MS gradients on a high-performance LTQ Orbitap Velos mass spectrometer, where all tandem mass spectra were recorded in the orbitrap analyser with high-resolution using the HCD technology. All LC-MS/MS raw files were processed together, peptide sequences were identified by Mascot and phosphoproteins were quantified using the MaxQuant software suite's label-free algorithm based on peptide extracted ion chromatograms. All raw files and annotated MS/MS spectra are provided as a resource (see Supplementary Data 1 ). In total, 876,203 high-resolution HCD-MS/MS events were collected of which 43% were identified with high confidence, which resulted in 28,733 unique phosphopeptides corresponding to 31,480 phosphorylation sites from 7,280 proteins. Tables with all identified phosphoproteins and phosphopeptides are provided in Supplementary Data 1 , 2 , 4 , and evaluation of the high-quality MS data is shown in Supplementary Fig. S1 . Furthermore, we have set up a web-accesible MySQL database named the CPR PTM Resource containing all identified phosphoproteins making it easy to search for identified phosphorylation sites on any given protein of interest: http://cpr1.sund.ku.dk/cgi-bin/PTM.pl . The confidence of phosphorylation site localization was evaluated for each site on every phosphopeptide and for annotation of a specific phosphorylation site a localization score ≥75% combined with a ΔPTM ≥5 was required. More than 70% of the sites we identified localized to a specific amino acid with a median localization score >99.9%. Thus, the combination of an efficient protein extraction procedure with high-accuracy mass spectrometric measurements allowed us to identify a large number of phosphorylation sites in a very limited time frame. The method outlined makes it possible to determine a tissue phosphoproteome in less than 2 days. 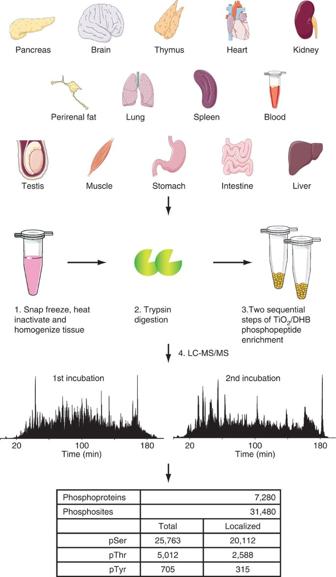Figure 1: Workflow for phosphoproteome analysis of rat tissue. A total of 14 different tissues were isolated from four male rats, followed by snap freezing, homogenization and solubilization of the tissues. For each tissue, 10 mg of protein was subjected to tryptic digestion, succeeded by duplicate steps of phosphopeptide enrichments using titanium dioxide beads. Both enrichments were analysed by high-resolution LC-MS/MS yielding a total of 31,480 phosphorylation sites. Figure 1: Workflow for phosphoproteome analysis of rat tissue. A total of 14 different tissues were isolated from four male rats, followed by snap freezing, homogenization and solubilization of the tissues. For each tissue, 10 mg of protein was subjected to tryptic digestion, succeeded by duplicate steps of phosphopeptide enrichments using titanium dioxide beads. Both enrichments were analysed by high-resolution LC-MS/MS yielding a total of 31,480 phosphorylation sites. Full size image Phosphoprotein expression pattern across tissues We first focused on the phosphoproteins identified in each LC-MS run and used normalized phosphoprotein intensities derived from summation of measured phosphopeptide extracted ion chromatograms to perform a comparative analysis. Hierarchical cluster analysis visualizes the experimental specificity and reproducibility ( Fig. 2a ). Reassuringly, the duplicate enrichments from each tissue cluster together, as does functionally related tissues, as for instance heart and muscle and the three brain regions investigated. Phosphoproteins are colour coded according to their MS signal intensities, which is a relative measure for protein abundance [30] , [31] , and the highlighted yellow areas thus indicate that the majority of tissues have abundant expression of a specific cluster of phosphoproteins. It is evident that the identified phosphoproteins vary in expression pattern as well as in phosphorylation site abundance among the tissues reflecting the physiological differences of the tissues. A few clusters of phosphoproteins are present in all tissues investigated, which is the pattern expected for instance for house-keeping proteins. Only few phosphoproteins identified in blood are also identified in other tissues, illustrating that our perfusion of the animals during euthanization was effective. The total number of phosphoproteins identified from each of the two enrichment steps is comparable within each tissue, but a slight gain in coverage is obtained with the second incubation resulting in an increased total number of phopshoproteins when merging the two data sets ( Fig. 2b ). For each tissue, the duplicate enrichments yield reproducible normalized phophopeptide intensity results with Pearson correlation coefficients in the range 0.77< R <0.90 (see Supplementary Figs S2–S6 ), which indicates that the technical reproducibility is high and that the detected heterogeneity in numbers of phosphoproteins per tissue reflects a true biological variation. The obtained clustering profile of phosphoprotein expression underscores the robustness of the method and gene ontology (GO) enrichment analysis further confirms this. GO term analysis of tissue-specific phosphoproteins reveal that these are indeed proteins with known tissue-specific roles, as for instance neuronal signalling regulation in brain and muscle contraction regulation in muscle and heart ( Supplementary Fig. S7 ). Conversely, phosphoproteins found in all tissues are proteins known to be important for all cell types, as for instance RNA processes and transcription. 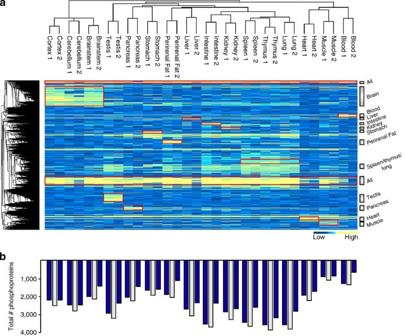Figure 2: Tissue distribution of phosphoproteins. (a) Hierarchical clustering of phosphoproteins and tissues based on label-free quantification of protein intensities from both enrichment steps (1 and 2). Low-intensity phosphoproteins are depicted in blue and high-intensity phosphoproteins are depicted in yellow. Red boxes highlight clusters of phosphoproteins that are either specific to a certain tissue or present in all tissues. (b) Histograms depicting the total number of phosphoproteins identified from each of the two enrichment steps (shown in blue) as well as the total number of phosphoproteins identified in each tissue obtained from merging the data from the two enrichment steps (shown in grey). Figure 2: Tissue distribution of phosphoproteins. ( a ) Hierarchical clustering of phosphoproteins and tissues based on label-free quantification of protein intensities from both enrichment steps (1 and 2). Low-intensity phosphoproteins are depicted in blue and high-intensity phosphoproteins are depicted in yellow. Red boxes highlight clusters of phosphoproteins that are either specific to a certain tissue or present in all tissues. ( b ) Histograms depicting the total number of phosphoproteins identified from each of the two enrichment steps (shown in blue) as well as the total number of phosphoproteins identified in each tissue obtained from merging the data from the two enrichment steps (shown in grey). Full size image Tissue-specific interaction networks of phosphoproteins To analyse the functions of the tissue-specific phosphoproteins further, we probed their molecular networks in silico . Such analyses are relevant as protein interaction networks with tissue resolution are valuable resources for deciphering and understanding the specific molecular systems driving pathological processes [32] , [33] . For each of the 14 tissues, we generated protein interaction networks using the tissue-specific phosphoproteins as seeds. Direct protein interactions, and indirect interactions through common interaction partners, were identified using a previously described database of quality controlled predicted and measured protein interaction data [32] , [34] , [35] . The data quality thresholds were optimized by permutation tests, and a network-building algorithm [35] , [36] was applied to build 14 protein interaction networks with tissue resolution. Eight of the fourteen networks interact significantly (1.0e-5 ≤adj. P ≤0.049, adjusted for multiple testing by Bonferroni correction, Supplementary Data 5 ), indicating that tissue-specific phosphoproteins have a strong tendency to directly interact, or are part of connected tissue-specific pathways. All networks are available in flat file format and in Cytoscape session format as a user-friendly community resource from http://cpr1.sund.ku.dk/cgi-bin/PTM.pl (see Supplementary Data 2 ). An example of a tissue-specific phosphoprotein network is shown in Fig. 3 , which illustrates a network based on phosphoproteins specifically identified in blood. By manual curation the network was found to consist of relevant functional clusters, such as coagulation, Kell blood group glycoprotein complex, haemoglobin and haem biosynthesis, inflammatory responses, immune regulation, and albumin-mediated transport. Our blood phosphoproteome is currently the largest phosphorylation data set measured from blood samples, and the protein interaction network expands our current understanding of the functional roles of phosphorylated proteins in blood [37] . 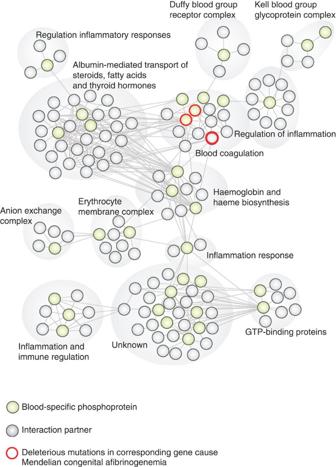Figure 3: Blood-specific phosphoprotein network. Protein interaction network based on phosphoproteins specifically identified in blood (green nodes) and expanded to include direct interaction partners (grey nodes). Protein clusters obviously relevant to blood biology, such as coagulation, Kell blood group glycoprotein complex, haemoglobin and haem biosynthesis, inflammatory responses, immune regulation and albumin-mediated transport, are highlighted. The network is available as a Cytoscape session file including accession numbers and protein names for all proteins in the network athttp://cpr1.sund.ku.dk/cgi-bin/PTM.pl. Figure 3: Blood-specific phosphoprotein network. Protein interaction network based on phosphoproteins specifically identified in blood (green nodes) and expanded to include direct interaction partners (grey nodes). Protein clusters obviously relevant to blood biology, such as coagulation, Kell blood group glycoprotein complex, haemoglobin and haem biosynthesis, inflammatory responses, immune regulation and albumin-mediated transport, are highlighted. The network is available as a Cytoscape session file including accession numbers and protein names for all proteins in the network at http://cpr1.sund.ku.dk/cgi-bin/PTM.pl . Full size image Tissue-specific versus globally expressed phosphoproteins A larger proportion of the identified phosphoproteins are tissue specific than globally expressed ( Fig. 4a ), with 11.4% of the identified phosphoproteins being found in one tissue only and 5.4% being found in all tissues. To investigate global patterns for the biological roles of the tissue-specific versus the globally expressed phosphoproteins, we made a GO term analysis comparing phosphoproteins found either in a single tissue or in all tissues to all other identified phosphoproteins ( Fig. 4b ). Globally expressed phosphoproteins are enriched for cytoplasmic and nuclear proteins involved in RNA processes, whereas tissue-specific phosphoproteins are enriched for plasma membrane proteins involved in ion transport and receptor-triggered signalling events. These findings are consistent with our current understanding that a large fraction of intracellular components are generic among cells, whereas specific cell types predominantly differ in the composition of proteins they expose at the plasma membrane [38] . Although we identify tissue-specific phosphoproteins in all tissues, we observe a significantly higher number of tissue-specific phosphoproteins in brain and testis compared with the other tissues investigated ( Supplementary Fig. S8 ), which is also consistent with data reported from mouse tissues [20] . This finding converges well with the GO term analysis in the sense that brain is expected to be the tissue investigated with the most diverse expression of ion channels and receptors and testis expresses many tissue-specific proteins. 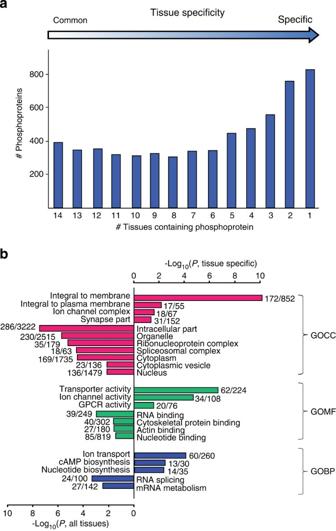Figure 4: Tissue specificity of phosphoproteins. (a) Histogram depicting the number of phosphoproteins identified in 1 to 14 tissues. (b) Phosphoproteins identified in one tissue are classified as tissue specific, whereas those identified in 14 tissues are classified as global. GO term analysis were made for tissue specific as well as global phosphoproteins. TheP-values for over-representation in either of the two categories were calculated with the Wilcoxin–Mann–Whitney test and a Benjamini–Hochberg false discovery rate test was applied to account for multiple testing. Enriched GO terms for cellular component (CC), molecular function (MF) and biological process (BP) are shown. The numbers next to each bar indicate how many proteins form basis for any given term, and how many of those are found among the enriched fraction. Figure 4: Tissue specificity of phosphoproteins. ( a ) Histogram depicting the number of phosphoproteins identified in 1 to 14 tissues. ( b ) Phosphoproteins identified in one tissue are classified as tissue specific, whereas those identified in 14 tissues are classified as global. GO term analysis were made for tissue specific as well as global phosphoproteins. The P -values for over-representation in either of the two categories were calculated with the Wilcoxin–Mann–Whitney test and a Benjamini–Hochberg false discovery rate test was applied to account for multiple testing. Enriched GO terms for cellular component (CC), molecular function (MF) and biological process (BP) are shown. The numbers next to each bar indicate how many proteins form basis for any given term, and how many of those are found among the enriched fraction. Full size image To estimate whether the map of rodent protein phosphorylation sites is comprehensive, we merged the rat data set presented here with the recently published mouse phosphoproteome data set [20] . At the protein level, we find 51.5% overlap between the phosphoproteins reported here, and those reported for the mouse, and at the site level the overlap is 23.2% ( Supplementary Fig. S9 ), thus indicating that the map is not yet comprehensive. Merging the two data sets result in a total of 9,287 rodent phosphoproteins harbouring an impressive 54,755 phosphorylation sites. This shows that phosphorylation is a post-translation modification with even more widespread impact on rodent proteins than previously estimated. Tissue distribution of specific phosphorylation sites In total, 23,415 of the identified phosphorylations can be localized to a specific residue using combined cut-off values of localization probability ≥0.75 and ΔPTM score ≥5, as previously described [16] . For each tissue, we investigated the relative abundance of phosphorylation sites of serine, threonine and tyrosine residues, and on average we find that serines account for 88.1%, threonines for 11.4% and tyrosines for 1.5% of all phosphorylation sites ( Fig. 5a ), which is consistent with previously published observations [16] , [20] . As a number of serine/threonine protein kinases are targeting specific sequence motifs, we used our data to evaluate the relative involvement of these kinases across tissues ( Fig. 5b ). As expected, we observe that basophilic kinases (PKA, PKD, AKT, CAMK2, AURORA and CHK) form a cluster, and that the relative sequence motif abundances of the majority of these kinases are comparable across most tissues. However, motifs matching those recognized by PKD and CHK kinases are relatively more abundant in stomach than in any other tissue, as are ATM motifs in blood and PLK motifs in skeletal muscle. Likewise, we find that CK2 and AKT motifs are abundant in pancreas, which is in line with reports on the involvement of the AKT signalling pathway in pancreatic cancer [3] , [39] , and CK2 involvement in insulin regulation of pancreatic β-cells [40] . It is also noticeable that the three different brain regions investigated exhibit similar patterns, which is consistent with our finding that cerebellum, cortex and brainstem appear very similar at the phosphoproteome level (also see Fig. 2a ). 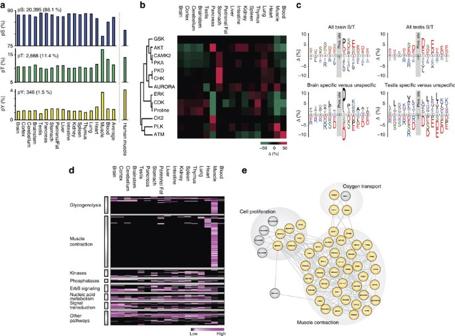Figure 5: Tissue distribution and amino-acid sequence features of localized phosphorylation sites. (a) Histograms depicting the percentages of serine, threonine and tyrosine phosphorylation sites identified in each rat tissue as well as in human skeletal muscle samples. The total number of S, T and Y phosphorylation sites across all tissues and their relative abundance in percent is stated above each histogram. (b) Heat map visualizing relative abundance of sequence motifs matching the indicated kinases from phosphopeptides identified in all tissues investigated. (c) Top: amino-acid sequence patterns for all S and T phosphorylation sites in brain and testis. Bottom: amino-acid sequence patterns for tissue-specific versus non-specific S and T phosphorylation sites for brain and testis. (d) Hierarchical cluster of pathway analysis of phosphotyrosine-containing proteins. (e) Protein–protein interaction network build from tyrosine-phosphorylated proteins identified in human skeletal muscle using InWeb shows that these proteins significantly interact with each other (Adj.P=2e-4, using a permuation test). The resulting network shows that tyrosine-phosphorylated proteins collaborate in muscle contraction, oxygen transport and cell proliferation to carry out physiological processes relevant to the tissue in question. The input proteins from human skeletal muscle are depicted as yellow spheres, whereas interacting proteins reported in the literature are depicted as grey spheres. Figure 5: Tissue distribution and amino-acid sequence features of localized phosphorylation sites. ( a ) Histograms depicting the percentages of serine, threonine and tyrosine phosphorylation sites identified in each rat tissue as well as in human skeletal muscle samples. The total number of S, T and Y phosphorylation sites across all tissues and their relative abundance in percent is stated above each histogram. ( b ) Heat map visualizing relative abundance of sequence motifs matching the indicated kinases from phosphopeptides identified in all tissues investigated. ( c ) Top: amino-acid sequence patterns for all S and T phosphorylation sites in brain and testis. Bottom: amino-acid sequence patterns for tissue-specific versus non-specific S and T phosphorylation sites for brain and testis. ( d ) Hierarchical cluster of pathway analysis of phosphotyrosine-containing proteins. ( e ) Protein–protein interaction network build from tyrosine-phosphorylated proteins identified in human skeletal muscle using InWeb shows that these proteins significantly interact with each other (Adj. P =2e-4, using a permuation test). The resulting network shows that tyrosine-phosphorylated proteins collaborate in muscle contraction, oxygen transport and cell proliferation to carry out physiological processes relevant to the tissue in question. The input proteins from human skeletal muscle are depicted as yellow spheres, whereas interacting proteins reported in the literature are depicted as grey spheres. Full size image As brain and testis have the greatest number of tissue-specific phosphoproteins, we investigated if there were any particular sequence motifs characteristic for the amino-acid sequences flanking the serine and threonines residues phosphorylated in brain or testis ( Fig. 5c ). From the visualized consensus motifs, it is evident that proline-directed phosphorylation is prominent in brain tissue but not in testis, whereas acidophilic kinase directed phosphorylation, for example, CK2, is pronounced in brain as well as testis. We next analyzed the amino-acid sequences flanking tissue-specific phosphorylation sites versus the phosphorylation sites found in other tissues for brain and testis, respectively. We find a strong signal for proline-directed phosphorylation for brain-specific phosphorylation sites, and for both tissues we observe that the CK2 substrate phosphorylation sites are not tissue specific. It thus appears that CK2-mediated phosphorylation in brain and testis is involved in regulation of proteins that are part of the general cellular machinery, whereas proline-directed phosphorylation occurs on proteins characteristic for brain tissue. Phosphorylation pattern in rat and human skeletal muscle When analyzing the distribution of S, T and Y phosphorylation sites across tissues, it became evident that the only tissue exhibiting a different pattern compared with all other tissues was skeletal muscle ( Fig. 5a ). In rat muscle, we found phosphorylation of tyrosine residues to account for 3.9% of all phosphorylations, which is a significant over-representation compared with the total average of 1.5% ( P <1.1e-8). Likewise, threonine sites account for 17.1% versus the tissue average of 11.4%. To investigate whether this pattern is a general trend of physiological relevance, we decided to study the phosphorylation pattern in human skeletal muscle samples. We analysed skeletal muscle biopsies taken from three healthy male subjects, and investigated the phosphoproteomes from these according to the same protocol as for the rat tissues (all identified phosphoproteins and phosphopeptides are provided in Supplementary Data 6 ). The human skeletal muscle phosphoproteomes resemble the phosphoproteome from rat skeletal muscle (see Supplementary Fig. S10a–b ), and our results from human muscle confirm the trend observed in rat muscle. In human skeletal muscle, tyrosine phosphorylation account for 4.3% and threonine for 14.2% of all phosphorylations ( Fig. 5a ). When analysing the sequence patterns flanking the serine and threonine phosphorylations identified in rat or human skeletal muscle samples and comparing these to the sequences found in all other tissues, we, as expected, find that threonine phosphorylations are over-represented, but we also find that proline-directed phosphorylation is greatly under-represented in muscle compared with all other tissues. When we compare the muscle-specific serine or threonine phosphorylation sites against the sites that are also found in other tissues, we again, as in brain and testis, find that CK2-mediated phosphorylation is over-represented for the sites that are not tissue-specific. For the muscle-specific phosphorylation sites there are no apparent consensus sequence, but there seems to be a preference for lysine and hydrophobic residues flanking the phosphorylation site ( Supplementary Fig. S10c ). To investigate the physiology underlying the over-representation of phosphotyrosines in muscle tissue compared with all other tissues, we next analysed all identified proteins carrying tyrosine phosphorylations in rat tissues with regards to their involvement in biological processes. As evident from the hierarchical clustering figure presented in Fig. 5d there are two major processes contributing to the different phosphotyrosine pattern of muscle tissue, namely glycogenolysis and muscle contraction. Although muscle contraction is also a crucial part of cardiac function, the majority of phosphotyrosines involved in skeletal muscle contraction are not present in the heart and vice versa. To investigate whether proteins involved in muscle contraction in human skeletal muscle are also tyrosine phosphorylated, we next investigated protein–protein interaction networks of tyrosine-phosphorylated proteins identified in human skeletal muscle biopsies ( Fig. 5e ). As evident from the figure proteins involved in the contractile machinery are indeed tyrosine phosphorylated. Receptor tyrosine kinases are the major class of enzymes responsible for tyrosine phosphorylation in mammalian cells [41] , but we do not identify any receptor tyrosine kinases in the skeletal muscle samples. However, we do identify tyrosine-phosphorylated peptides from the activation loop (T-loop) of the kinase domains of both the cytoplasmic tyrosine kinases Yes/Src/Lck/Fyn (LIEDNEYpTAR) and Lyn/Hck (VIEDNEYpTAR) as well as of the dual-specificity tyrosine-regulated kinase DYRK1A/B (IYQYpIQSR and IYQYpIQSpR). Both of these kinase classes phosphorylate their substrates on tyrosine residues and phosphorylation of their activation loops are a proxy for their activation state in the skeletal muscle [42] , which suggest that these kinases are involved in regulation of the skeletal muscle tyrosine phosphoproteome. For the human skeletal muscle samples, we also identify multiple haemoglobin subunits with tyrosine phosphorylations, which can be explained by the lack of perfusion in the human muscle sample preparation. To further investigate the metabolic process with high levels of phosphotyrosines involving glucose metabolism, we delineated the pathway of glycogenolysis in Fig. 6 . Glycogenolysis predominantly occurs in muscle cells as a means to produce energy, and it is highly regulated dependent on the metabolic state. However, it also occurs in the liver where glucose is produced and released into the blood to maintain adequate glucose levels. To survey differences in glycogenolysis among muscle and liver tissues, we highlighted the phosphoproteins involved in the pathway in the two tissues along with the phosphorylation sites detected. As evident from the figure, the phosphoproteins involved in the pathway were well covered for both tissues, but we only identified a large proportion of tyrosine-phosphorylated proteins in muscle. Again, the involvement of phosphotyrosines appears to be a common phenomenon of physiological relevance, as it was observed in rat as well as in human skeletal muscle. This is also supported by the recent findings of tyrosine phosphorylation sites as critical regulators of glycolytic pathway enzymes like lactate dehydrogenase A [43] and pyruvate dehydrogenase kinase 1 (ref. 44 ) for cancer cell metabolism. As most signalling networks rely on sequential and coordinated phosphorylation of specific pathway proteins, it is intriguing that tyrosine phosphorylation is much more prevalent in muscle compared with liver, thus suggesting that glycogenolysis is likely regulated by tyrosine kinases in muscle, whereas this is not the case in liver. 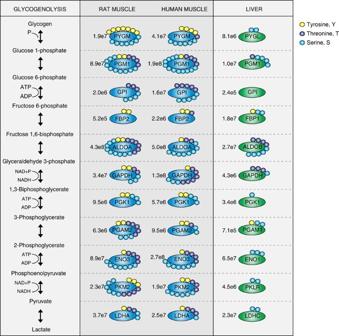Figure 6: Muscle and liver glycogenolysis. The chemical pathway for glycogenolysis is shown as are the phosphorylated enzymes involved in each of the steps identified in rat or human skeletal muscle (left) or in liver (right). The protein isoforms with the greatest number of identified phosphorylation sites were chosen for visualization. The number of phosphorylation sites on each of the proteins is indicated by small circles that are colour coded according to the amino acid phosphorylated with yellow for tyrosine, purple for threonine and blue for serine. The normalized protein intensity count is provided next to each protein. Figure 6: Muscle and liver glycogenolysis. The chemical pathway for glycogenolysis is shown as are the phosphorylated enzymes involved in each of the steps identified in rat or human skeletal muscle (left) or in liver (right). The protein isoforms with the greatest number of identified phosphorylation sites were chosen for visualization. The number of phosphorylation sites on each of the proteins is indicated by small circles that are colour coded according to the amino acid phosphorylated with yellow for tyrosine, purple for threonine and blue for serine. The normalized protein intensity count is provided next to each protein. Full size image Proline-directed kinases phosphorylate transcription factors Proline-directed kinases, such as CDKs and MAPKs, have some of the best-described amino-acid sequence motifs, and thus we next focused on all the proline-mediated phosphorylation sites we have identified. We compared the presence of proline-mediated phosphorylation sites among different cellular compartments, focusing on the extracellular space, the plasma membrane, the cytoplasm, the endoplasmic reticulum and golgi as well as the nucleus. The highest abundance of proline-mediated phosphorylation sites is identified in the nucleus, where we observe both the greatest prevalence frequency and the greatest number of proline-mediated phosphorylation sites ( Fig. 7a ). To investigate the biological underpinnings for this, we focused on two classes of proteins particular for the nucleus, namely protein kinases and transcription factors ( Fig. 7b ). We used a similar approach as presented by Rigbolt et al . [45] to extract transcription factors from our data set based on annotated DNA-binding protein domains (HLH, HMG-box, bZIP, Forkhead and Homeobox). The prevalence of proline-directed phosphorylation sites of protein kinases is similar to that of all identified phosphorylation sites, whereas the prevalence is significantly greater for transcription factors. The fraction of phosphorylation sites that are proline-mediated becomes even greater when we focus on tissue-specific phosphorylation sites on transcription factors. Analysing the amino-acid sequences of the proline-mediated phosphorylation sites in the nucleus, it is apparent that these are generally mediated by CDK kinases by conforming to the proline-directed motif with basophilic residues in the +2 or +3 position ( Fig. 7c ). However, analysing amino-acid sequences of all phosphorylation sites identified on transcription factors reveals an apparent MAP kinase sequence logo [P-X-S/T-P] ( Fig. 7d ), consistent with previous reports on widespread transcriptional regulation by MAP kinases [46] . Thus, in general proline-directed phosphorylation is highly abundant in the nucleus, and it is primarily mediated by CDK kinases, but proline-directed phosphorylation of transcription factors are mediated by MAP kinases. The tissue-specific proline-directed phosphorylation sites on transcription factors are listed in the table in Supplementary Fig. S11 . 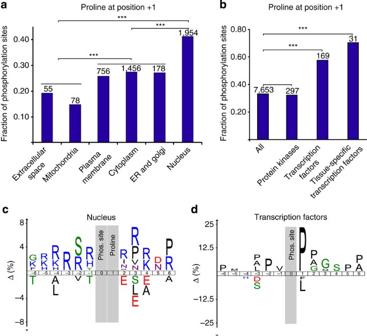Figure 7: Proline-directed phosphorylation. The fraction of localized phosphorylation sites that harbour a proline residue at the adjacent position +1 for six different cellular compartments (a) and for protein kinases and transcription factors (b) are depicted as histograms. The number of identified phosphorylation sites with a proline at position +1 for each category is indicated above the bars. Studentst-test, ***P>0.001. (c) Amino-acid sequence pattern for phosphorylation sites on nuclear proteins with a proline at position +1 versus phosphorylation sites with a proline at position +1 on all non-nuclear proteins. (d) Amino-acid sequence pattern for phosphorylation sites on transcription factors compared with all other phosphorylation sites. ER, endoplasmic reticulum. Figure 7: Proline-directed phosphorylation. The fraction of localized phosphorylation sites that harbour a proline residue at the adjacent position +1 for six different cellular compartments ( a ) and for protein kinases and transcription factors ( b ) are depicted as histograms. The number of identified phosphorylation sites with a proline at position +1 for each category is indicated above the bars. Students t -test, *** P >0.001. ( c ) Amino-acid sequence pattern for phosphorylation sites on nuclear proteins with a proline at position +1 versus phosphorylation sites with a proline at position +1 on all non-nuclear proteins. ( d ) Amino-acid sequence pattern for phosphorylation sites on transcription factors compared with all other phosphorylation sites. ER, endoplasmic reticulum. Full size image Here we show that an efficient method for tissue protein extraction in combination with phosphopeptide enrichment and high-resolution tandem MS can quantify an impressive amount of phosphopeptides and protein phosphorylation sites from tissue samples in a limited time. The method was validated by the clustering profile of the phosphopeptides in specific tissues and by reproducing the tyrosine phosphorylation pattern found in rat and human skeletal muscle samples. From a scientific perspective, the data set we report herein provides a useful resource for future hypothesis-driven exploration of tissue-specific variations in phosphorylation-mediated regulation of proteins; thereby also presenting the opportunity to identify new cellular targets for regulatory phosphorylation events. Furthermore, with the increasing evidence manifesting involvement of dysfunctional signalling cascades, not only in many types of cancer, but also in diabetes and neuropsychiatric disorders, the need for unravelling signalling cascades in the appropriate tissues are underscored. From the data presented it is evident that there are major differences in the phosphorylation patterns across tissues, and accordingly it is apparent that for understanding the molecular mechanisms underlying disease signalling pathways, it is crucial to investigate the components in the appropriate tissue with site specificity. To do this successfully, it is a prerequisite that reliable and comprehensive methods are developed that allow for such investigations. In the future, it will furthermore be beneficial if tissue samples from patients can be analysed as a mean to evaluate which medical treatment is most appropriate. From cancer patients, it is for instance known that there is great variation in how well the patients respond to different treatments, likely due to patient-specific differences in affected steps of the signalling pathways. As the method presented herein is a rapid procedure that only requires a few hours of LC-MS/MS analysis time per tissue, thus making it much simpler and time-preserving compared with previously presented methods, it provides a promising platform for standardizing screening of tissue phosphoproteomes. Sample preparation and peptide extraction The study was carried out following approved national regulations in Denmark and with animal experimental licence granted by the Animal Experiments Inspectorate, Ministry of Justice, Denmark. Four Sprague Dawley rats (Crl:SD, male, 350 g , Charles River, Germany) were anaesthetized with isoflurane and perfused (1½ min, 30 ml min −1 ) with isotonic saline-containing protease inhibitors (0.120 mM EDTA, 14 μM aprotinin, 0.3 nM valine-pyrrolidide and, Roche Complete Protease Inhibitor tablets (Roche), pH=7.4) before being decapitated. The organs were quickly dissected, and except for the brain they were all snap frozen in 2-methylbutane followed by heat inactivation (Denator T1 Heat Stabilizor, Denator, Gothenburg, Sweden). After dissection, the brain was heated to 95 °C (by a Denator T1 Heat Stabilizor), subdissected into cerebellum, cortex and brainstem. Non-heparinized trunk blood was collected from another group of four rats by decapitation. Human muscle biopsies were obtained from the musculus vastus lateralis in three healthy volunteers during resting conditions with a needle modified for suction under local anaesthetics using the Bergström technique [47] . The study-part including human volunteers conformed to the Helsinki II declaration and was approved by the relevant local ethics committee (Ethical approval number H-A-2009-016 for Region Hovedstaden, Denmark). The biopsy specimens were rapidly transferred to liquid nitrogen (within 5 s), and thereafter stored at −80 °C until analysed. The tissues were transferred to a urea solution containing phosphatase inhibitors (6 M urea/2 M thiourea, 10 mM HEPES, 1 mM ortho-vanadate, 5 mM sodium flouride, 5 mM β-glycerophosphate, pH=8.0) in 5 μl extraction buffer per mg tissue (wet weight) and homogenized by ceramic beads using 1–6 homogenization steps of 20 s at 5,000 r.p.m. (Precellys 24, Bertin Technologies, France) followed by micro-tip sonication on ice. The homogenized samples were centrifuged (20 min, 16,000 g , 4 °C) and the supernatants were retrieved. Protein digestion Samples were reduced (final concentration 1 mM dithiothreitol, 750 r.p.m., 30 min), and alkylated (final concentration 5.5 mM chloroacetamide, 750 r.p.m., 20 min in darkness). Protein concentrations were measured (Quick Start Bradford Dye Reagent X1, Bio-Rad) and 10 mg protein per tissue was digested with 50 μg endoproteinase Lys-C (Wako) (750 r.p.m., 3 h). The samples were diluted with 25 mM ammonium bi-carbonate to lower the urea concentration below 2 M, and then further digested with 50 μg modified trypsin (Sequencing grade, Promega; 750 r.p.m., 8 h). Trypsin digestion was quenched by lowering pH ~2 with trifluoroacetic acid (TFA). Samples were centrifuged (20 min, 16,000 g ) and supernatants were desalted and concentrated on Sep-Pack C 18 Cartridges (Waters). Enrichment of phosphopeptides The phosphopeptides in the samples were enriched using Titanium dioxide (TiO 2 ) beads essentially as described in Olsen et al . [16] A stock solution of 20 mg TiO 2 beads (GL Sciences, Japan) per 100 μl 2,5-dihydroxybenzoic acid (DHB; 0.02 g DHB per ml 80% acetonitrile (MeCN), 0.5% acetic acid (AcOH)) were mixed for 15 min, 5 μl of this was added to the samples, which were then incubated with gentle rotation for 15 min. The TiO 2 beads were quickly spun down and the supernatants were transferred to new Eppendorf tubes and incubated with a second round of TiO 2 beads as described above. The beads were washed with 100 μl of 5 mM KH 2 PO 4 , 30% MeCN, 350 mM KCl followed by 100 μl of 40% MeCN, 0.5% AcOH, 0.05% TFA and then re-suspended in 50 μl of 80% MeCN, 0.5% AcOH. The beads were loaded onto in-house packed C 8 STAGE tips in 200 μl pipette tips preconditioned with 80% MeCN, 0.5% AcOH and washed once with the same buffer, and eluted with 2×10 μl 5% ammonia and 2×10 μl 10% ammonia, 25% MeCN. Ammonia and organic solvents were evaporated using a vacuum centrifuge, and the peptides were acidified in 1% TFA, 5% MeCN and loaded onto in-house packed C 18 STAGE tips [48] preconditioned with 20 μl MeOH, 20 μl 80% MeCN, 0.5% AcOH, 2×20 μl 1% TFA, 3% MeCN. Stage tips were washed with 2×20 μl of 8% MeCN, 0.5% AcOH, and 1×50 μl of 0.5% AcOH. LC-MS/MS analysis Peptides were eluted into 96-well microtiter plates with 2×10 μl of 40% MeCN, 0.5% AcOH, organic solvents were removed in a vacuum centrifuge, and the peptides were reconstituted in 2% MeCN, 0.5% AcOH, 0.1% TFA. A volume of 5 μl of this eluate was analyzed by online reversed-phase C 18 nanoscale liquid chromatography tandem MS on an LTQ-Orbitrap Velos mass spectrometer (Thermo Electron, Bremen, Germany) using a top10 HCD fragmentation method as described previously [27] . The LC-MS analysis was performed with a nanoflow Easy–nLC system (Proxeon Biosystems, Odense, Denmark) connected through a nano-electrospray ion source to the mass spectrometer. Peptides were separated by a linear gradient of MeCN in 0.5% acetic acid for 180 min in a 15-cm fused-silica emitter in-house packed with reversed-phase ReproSil-Pur C 18 -AQ 3 μm resin (Dr Maisch GmbH, Ammerbuch-Entringen, Germany). Full-scan MS spectra were acquired at a target value of 1e6 and a resolution of 30,000, and the HCD-MS/MS spectra were recorded at a target value of 5e4 and with resolution of 7,500 using a normalized collision energy of 40%. Phosphopeptide quantification and identification Raw MS files were processed using the MaxQuant software [49] (ver.1. 0.14.7, Max-Planck Institute of Biochemistry, Department of Proteomics and Signal Transduction, Munich) by which the precursor MS signal intensities were determined and HCD-MS/MS spectra were de isotoped and filtered such that only the ten most abundant fragments per 100- m / z range were retained. Phosphoproteins were identified using the Mascot search algorithm ( http://www.matrixscience.com ) by searching all MS/MS spectra against a concatenated forward/reversed version of rat and mouse International Protein Index v.3.37 protein sequence database supplemented with protein sequences of common observed contaminants such as human keratins and porcine trypsin. The HCD-MS/MS spectra were searched with fixed modification of Carbamidomethyl-Cysteine and we allowed for variable modifications of oxidation (M), acetylation (protein N-term), Gln->pyro-Glu, and phosphorylation (STY). Search parameters were set to an initial precursor ion tolerance of 7 p.p.m., MS/MS tolerance at 0.02 Da and requiring strict tryptic specificity with a maximum of two missed cleavages. Label-free peptide quantification and validation was performed in the MaxQuant software suite [49] , [50] . Phosphopeptides were filtered based on Mascot score, PTM (Andromeda) score [51] , precursor mass accuracy, peptide length and summed protein score to achieve an estimated false discovery rate <0.01 based on the forward and reversed identifications [52] . The minimum required peptide length was set to six amino acids. We required a minimum Mascot score of 10 and a minimum Andromeda score of 25. Data analysis and presentation Data analysis was done using Microsoft Office Excel and Perseus [53] (Max-Planck Institute of Biochemistry, Department of Proteomics and Signal Transduction, Munich) software. Tissue figures were produced using Servier Medical Art ( http://www.servier.com ). Hierarchical clustering was performed in Persues using Euclidian distance and average linkage clustering. GO enrichment analysis was alike performed in Perseus, either for a cluster of tissue-specific proteins or for phosphoproteins present in either one or all tissues. The whole quantified phosphoprotein data set was used as reference data set and P -values were calculated using the Benjamini–Hochberg method. Linear kinase motif analysis We analysed the frequency of particular amino acids in the proximity of phosphorylation sites by looking for specific kinase phosphorylation motifs. To avoid noise in the analysis from motifs without unambiguously assigned phosphorylation sites, we used only sites with a localization probability >0.75 and ΔPTM score >5 (class 1) for the analysis. To search for over-represented motifs, we used sequence windows of ±6 residues adjacent to all serine and threonine phosphorylation sites and matched these against ten known linear protein kinase motifs ( http://www.phosida.com ) representing PKA, AKT, PKD, CAMK2, CHEK, CK2, PLK, CDK, ERK and ATM/ATR kinases, as well as proline-directed substrate sites. The frequency of all kinase motifs were extracted for each tissue individually and compared with the median occurrence in all 14 tissues. To identify tissue enriched as well as under-represented motifs, we calculated the percentage difference between the individual tissues and the median occurrence for each kinase motif and clustered this matrix in Perseus using correlation-based two-way hierarchical clustering. Sequence pattern analysis We performed sequence pattern analysis using iceLogo [54] with percentage difference as scoring system and a P -value cut-off of 0.05. For details see Supplementary Data 3 . CPR PTM resource The CPR PTM Resource ( http://cpr1.sund.ku.dk/cgi-bin/PTM.pl ) is a web-based data repository that integrates all of the high-confidence in-vivo post-translational modifications sites such as site-specific phosphorylation that we have identified by MS-based proteomics in different tissue samples from various species. It is based on a MySQL database and developed with the Perl/CGI language. Modified proteins can be visualized based on their Uniprot identifiers. For each modified site in a protein, we list matching kinase motifs and use the Reflect ( http://reflect.cbs.dtu.dk/index.html ) service to add additional information about the modified proteins. Selected screen shots from the website are displayed in Supplementary Fig. S12 . Protein–protein interaction networks Protein–protein interaction networks were built using a previously described up to date interaction network of quality controlled predicted and measured human protein interactions (InWeb, Lage et al . [34] ). Detailed description is provided in Supplementary Data 4 . How to cite this article: Lundby, A. et al . Quantitative maps of protein phosphorylation sites across 14 different rat organs and tissues. Nat. Commun. 3:876 doi: 10.1038/ncomms1871 (2012).